Complete sequences ofSchizosaccharomyces pombesubtelomeres reveal multiple patterns of genome variation Genome sequences have been determined for many model organisms; however, repetitive regions such as centromeres, telomeres, and subtelomeres have not yet been sequenced completely. Here, we report the complete sequences of subtelomeric homologous ( SH ) regions of the fission yeast Schizosaccharomyces pombe . We overcame technical difficulties to obtain subtelomeric repetitive sequences by constructing strains that possess single SH regions of a standard laboratory strain. In addition, some natural isolates of S. pombe were analyzed using previous sequencing data. Whole sequences of SH regions revealed that each SH region consists of two distinct parts with mosaics of multiple common segments or blocks showing high variation among subtelomeres and strains. Subtelomere regions show relatively high frequency of nucleotide variations among strains compared with the other chromosomal regions. Furthermore, we identified subtelomeric RecQ-type helicase genes, tlh3 and tlh4 , which add to the already known tlh1 and tlh2 , and found that the tlh1–4 genes show high sequence variation with missense mutations, insertions, and deletions but no severe effects on their RNA expression. Our results indicate that SH sequences are highly polymorphic and hot spots for genome variation. These features of subtelomeres may have contributed to genome diversity and, conversely, various diseases. Genomic DNA sequences provide fundamental information for biological study. The genomes of model organisms, such as Saccharomyces cerevisiae ( S. cerevisiae ) [1] , Schizosaccharomyces pombe ( S. pombe ) [2] , Caenorhabditis elegans [3] , Drosophila melanogaster [4] , Arabidopsis thaliana [5] , and Homo sapiens [6] , [7] , [8] , have been sequenced in the past two decades, and most parts of these sequences have been reported. However, sequencing of long repetitive regions has not been completed because of technical difficulties in sequencing and chromosome allocation of such regions, as well as frequent occurrence of mutations and structural changes caused by chromosome rearrangements, such as recombination, translocation, chromosome breakage, and fusion [9] , [10] , [11] , [12] , [13] . Incomplete genomic DNA information can lead to inaccurate data in some experiments. For instance, we are unable to determine the precise chromatin localization of proteins in repetitive regions without actual DNA sequences. Evaluation of protein localization by chromatin immunoprecipitation assays involves PCR with sets of representative primers that target repetitive sequences or Southern blot analysis with representative probes. Chromatin localization values obtained using representative primers or probes merely show averages of all regions that have the target sequences, and they do not reflect actual patterns of chromatin association. Next-generation sequencers (NGSs) do not solve this problem if complete genome sequences are not provided. In addition, there may be uncharacterized genes in un-sequenced regions. Therefore, complete sequences of genomic DNA are crucial for accurate analyses and a deeper understanding of model organisms. Telomeres, which exist at chromosome ends and possess species-specific tandem repeat sequences, play crucial roles in several cellular activities required for cell survival, including protection of chromosome ends, length regulation of telomere-specific repeat DNA, and regulation of chromosome movements during mitosis and meiosis [14] , [15] , [16] , [17] . Subtelomeres, which are adjacent to telomeres, have sequences distinct from telomere repeats and generally contain multiple species-specific segments that share high similarity with other subtelomeres. In the budding yeast S. cerevisiae , the subtelomeres contain X and Y′ elements, the latter of which includes the open reading frame (ORF) of a helicase gene [18] . In humans, the subtelomeres are mosaics of ~50 types of common segments containing various ORFs, such as those for the DUX4 gene, which is related to facioscapulohumeral muscular dystrophy, and for the olfactory receptor family genes [9] , [19] , [20] . Although substantial knowledge of telomeres has accumulated, research on subtelomeres has progressed slowly compared with research on other chromosomal regions because of technical difficulties caused by long and repetitive nature of this region and partially unknown sequences. The fission yeast S. pombe is one of the most commonly used yeast model organisms for biological study. It preferentially proliferates as haploid in nutrient-rich media and possesses only three chromosomes (chromosome 1 [Ch1], 5.6 Mb; Ch2, 4.6 Mb; Ch3, 3.5 Mb), which enables the whole package of genetic analyses, such as screening for both dominant and recessive mutations, and generation of cells with circular chromosomes by deleting telomere DNA. S. pombe subtelomeres spanning ~100 kb are subdivided into two regions of ~50 kb each, the telomere-adjacent and telomere-distal regions (Fig. 1a ). The telomere-adjacent regions ( SH [ s ubtelomeric h omologous] regions) of subtelomeres contain SH sequences, which share high similarity (>90% identity) with at least one other subtelomere in S. pombe [21] and form heterochromatin structures [22] , [23] . This SH region is subdivided into two regions, the telomere-proximal SH-P and telomere-distal SH-D regions by their different features in 972 strains (Fig. 1a ; see below). In contrast, the SH- adjacent regions ( SU [ s ubtelomeric u nique] regions) share almost no sequence similarity with other subtelomeres, but exhibit common highly condensed chromatin structures called knobs [24] (Fig. 1a ). Because of high sequence similarity, it is very difficult to distinguish individual SH regions of subtelomeres at different chromosome ends and to assemble repetitive subtelomeric sequences accurately, even if we use latest NGSs. Therefore, parts of SH regions remain un-sequenced for 19 years after vast majority of the S. pombe genome sequence was reported ( S. pombe genome database, PomBase: http://www.PomBase.org/status/sequencing-status ) [2] (Fig. 1b ). Previously, parts of the four SH regions have been cloned and sequenced (pNSU series, see below) [25] ; however, they have not yet been allocated to specific subtelomeres (see PomBase). Fig. 1: Structures and previously unsequenced regions of subtelomeres in S. pombe 972 strain. a Schematic illustration of the structures of subtelomeres (~100 kb) of Ch1 and Ch2 in strain 972 . The SH region (~50 kb) shows high sequence identity (>90%) with other subtelomeres. Subtelomeric heterochromatin is formed around the SH region [21] . An SH sequence is composed of two characteristic regions, SH-P (~5 kb) and SH-D . In contrast, the SH -adjacent SU region (~50 kb) shows low sequence identities with other subtelomeres, but forms a highly condensed knob structure that is shared among them [24] . SA indicates a subtelomere-adjacent euchromatin region. b Schematic illustration of unsequenced regions of subtelomeres in Ch1 and Ch2 of strain 972 according to PomBase (indicated by orange boxes). Tel1L , tel1R , tel2L , and tel2R indicate telomeres at the left and right arms of Ch1 and those of Ch2, respectively. Subtel1L , subtel1R , subtel2L , and subtel2R indicate subtelomeres at the left and right arms of Ch1 and those of Ch2, respectively. Lengths of unsequenced regions are estimated based on the assumption that these SH sequences show high similarity with that of subtel2R of PomBase. Note that Ch3 is omitted in this panel (see Fig. 2a for the ends of Ch3 in strain 972 ). Full size image Construction of strains containing single SH regions of 972 To overcome the difficulty in allocating each SH sequence to a specific subtelomere, we constructed strains containing single SH regions of the standard S. pombe strain 972 ( h − ). Strain 972 used in this study (a derivative of the original 972 (ref. [26] )), which has not been crossed with other strains, possesses four SH sequences ( SH1L , SH1R , SH2L , and SH2R , as shown in Fig. 2a ) adjacent to the telomeres of Ch1 and Ch2, but no SH sequence in Ch3 (note that some descendent strains of 972 possess a partial (~16 kb-long) SH sequence adjacent to the telomeres of the left and/or right arms of Ch3; see Supplementary Fig. 1 ) [21] , [27] , [28] . We previously produced the SD5 ( S H d eletion 5) strain, in which all five SH regions that are located at both ends of Ch1 and Ch2, and the left end of Ch3 were replaced with a marker gene ( his7 + or ura4 + ) in a nonstandard strain JP1225 background [21] . Strain 972 was crossed with SD5 , and the first or second filial progeny were analyzed for the presence or absence of each SH region by pulse-field gel electrophoresis (PFGE) followed by Southern blotting (Fig. 2a–d ; also see “Methods” section). We screened for strains that exhibit a single band of telomere-associated sequence (TAS) [29] (i.e., SH ). We obtained strains that contain a single SH region of 972 and named them 972SD4[1 L +, 1 R +, 2 L +, or 2 R + ] , since they carry deletions of four SH regions in the original SD5 and one intact SH region from 972 . Each intact SH region in 972SD4 was named as 972SD4-SH1L , 972SD4-SH1R , 972SD4-SH2L , or 972SD4-SH2R . Fig. 2: Construction of 972SD4 strains containing a single SH region of strain 972 . a Construction strategy of 972SD4 strains. Pale green boxes, SH regions adjacent to telomeres; black boxes, marker genes ( his7 + or ura4 + ) that replaced SH regions [21] ; orange boxes, rDNA repeats; and red boxes, centromeres. Strains 972 and SD5 were crossed, and meiosis and sporulation (spore formation) were induced. Progeny with single SH regions were obtained. b Schematic illustration of telomere-containing NotI restriction fragments (shown in gray). Fragments L, I, M, and C contain SH1L , SH1R , SH2L , and SH2R , respectively. The size of each fragment is shown underneath. c Schematic illustration of the positions of DNA fragments detected by probes for telomeres and TAS (TAS1–3). Shown are the distances from telomeres in pNSU70. d Analyses of the chromosome end structures in 972SD4 strains. NotI-digested chromosomal DNAs of three independent strains of each 972SD4 were analyzed by PFGE followed by Southern blotting using telomere, TAS, or SPBCPT2R1.03 ORF probes. EtBr, ethidium bromide staining of the gel after PFGE. Note that SH1R lacks part of the SH region homologous to SPBCPT2R1.03 according to PomBase. Consistently, 972SD4[1 R + ] strains did not show an SPBCPT2R1.03 . signal (also see Fig. 5 ). These data were reproduced twice. Full size image Cloning and sequencing of SH-P regions From the data in PomBase, multiple common segments aligned in a mosaic pattern were expected for the SH-P region (see below). In order to accurately assemble such repetitive sequences, we amplified the SH-P region (~5 kb) in each 972SD4 by PCR and cloned into a vector. Partial deletion series of the SH-P fragments was constructed by digesting the plasmids with restriction enzymes followed by treatment with exo- and endo-nucleases. Re-circularized plasmids that carry the SH-P fragments with various lengths were sequenced using primers that anneal to the vector (Supplementary Fig. 2 , see “Methods” section). SH-P regions exhibit highly variable mosaic structures consisting of common segments We classified the sequences of SH-P regions of the 972SD4 strains, a part of SH2R in PomBase (PomBase- SH2R ), and insertions in the pNSU series in PomBase [25] into common segments (A–X) as follows. First, the sequences of SH-P regions were classified into common segments that meet the criteria of ≥ 50 bp and >95% identity using NCBI nucleotide BLAST (blastn) program (v2.10.0+, https://blast.ncbi.nlm.nih.gov/Blast.cgi ). Then, gaps between the segments were classified into additional segments that meet the criteria ≥14 bp and >95% identity. Segments were classified into variants (e.g., A1 and A2) that meet the criteria of 100% identity (Fig. 3a and Supplementary Fig. 3 ). To reduce the number of common segments, exceptional rules were applied for subtypes C (C1–3) and C′, E, E′, and E′′, K and K′, and S and S′, which contain different copies of several common sequence motifs that show 100% identities except for motifs in subtype C, c1–8 (Fig. 3b and Supplementary Fig. 3 ). SH-P regions in two independent strains (#1 and #2) of 972SD4[1 L + ] , 972SD4[1 R + ] , and 972SD4[2 L + ] exhibit 100% sequence identity, suggesting that no mutation or rearrangement have been introduced to the SH-P sequences of these 972SD4 strains during crossing, amplification by PCR, cloning using Escherichia coli ( E. coli ), and construction of serial deletion mutants. In contrast, two strains of 972SD4[2 R + ] contain different variants of segment D, D1 and D3, which show differences in two nucleotides, suggesting that the two point mutations at segment D and/or interchromosomal recombination have occurred in 972 or 972SD4[2 R + ] (Fig. 3a and Supplementary Fig. 3d ). Fig. 3: Highly variable SH-P regions consist of common segments in strain 972 . a Schematics of SH-P regions. The SH-P sequences were classified into common segments (A–X) and their variants (see Supplementary Fig. 3 for each sequence). SH-P regions of 972SD4 strains, a partial SH2R region in PomBase (PomBase- SH2R ), and SH-P regions of a pNSU series in PomBase are shown. The total length of each SH-P region is indicated. Note that 972SD4-SH1L , 972SD4-SH1R , and 972SD4-SH2L obtained from two independent 972SD4 strains (i.e., #1 and #2 clones) are identical, whereas 972SD4-SH2R #1 and #2 contain different variants D, D1 and D3. Black bars indicate relatively long regions that show the same segments and variants with those of pNSUs or PomBase- SH2R , whereas gray dotted lines indicate regions that show the same segments but different variants. b Subtypes of C, E, K, and S consist of common sequence motifs with different copy numbers. The boxes with the same color and pattern show 100% sequence identity. Segment C consists of three variants, C1–3, that are composed of homologous sequence motifs, c1–8, that show >82% identities with each other (see Supplementary Fig. 3c, c* for details). Full size image We found that none of the SH-P regions of 972SD4 show the same pattern in the alignment of segments to each other; however, two pairs of regions, 972SD4-SH1L and pNSU21/65, and 972SD4-SH2L and pNSU64, each exhibit the same segment patterns over the whole SH-P regions, suggesting the possibility that these pairs were derived from the same subtelomeres. However, the compositions of the C and D variants are different (C1 vs. C2 or C3, and D1 vs. D3; Fig. 3a , gray dotted lines). We found that segments C in 972SD4 strains are particularly different from those of pNSUs (Fig. 3a , gray dotted lines); i.e., variant C1 is the majority in the SH-P sequences of 972SD4 , whereas variant C2 is the majority in those of pNSUs. These data suggest that segment C is prone to mutation and recombination possibly due to its highly repetitive structure (Fig. 3b ). In contrast to 972SD4-SH1L and 972SD4-SH2L , 972SD4-SH1R and 972SD4-SH2R show combinations of pNSU patterns (Fig. 3a ). Moreover, subtypes E′′ and K′, and variant H2 are unique to 972SD4-SH1R among the SH-P sequences of 972SD4 and PomBase- 972 , suggesting that multiple times of mutation and recombination have occurred at 972SD4-SH1R . Surprisingly, 972SD4-SH2R exhibits a pattern different from a part of the PomBase -SH2R sequence; indeed, the pattern of PomBase -SH2R is found in a part of 972SD4-SH1L , implying that SH1L and SH2R have exchanged their chromosomal positions over repeated rounds of cell divisions. Although we identified several variants for each segment, these variants are not randomly combined, and partial sequences show the same alignments; for instance, there are two common alignments: P1-Q1-----V-Q3 (in 972SD4-SH1L , PomBase- SH2R , pNSU21/65, and pNSU70/77) and E-F2-----P3-Q3 (in 972SD4-SH2L , 972SD4-SH2R #1, 972SD4-SH2R #2, and pNSU64). Overall changes in the segment and variant compositions imply that SH-P regions are prone to nucleotide change and chromosome rearrangement. SH-P regions exhibit high variation in segmental arrangement among 972 strains and natural isolates of S. pombe To elucidate how SH-P regions have changed in the course of culturing or evolution, we next extracted uncharacterized sequences of the SH-P regions in various natural isolates of S. pombe in J. Bähler’s laboratory in UK (JB strains), using previous raw data by Tusso et al. (long-read sequencing using Nanopore MinION and PacBio RS II) [30] (Fig. 4a , see “Methods” section for details). Our analyses on chromosome configuration suggested that chromosome end fragment of Ch1R has been swapped with that of Ch2R in JB934 in comparison with 972 , as described previously (Supplementary Fig. 4 ) [30] . Although long-read sequencing data lack accuracy, we were able to analyze patterns of segments (A–X) and subtypes, but not at the variant level (see figure legends of Fig. 4 for details). Fig. 4: High variation in SH-P regions in diverse S. pombe strains. a Phylogenetic relationships among 972 and JB strains based on genome-wide sequences according to a previous study by Tusso et al. [30] . Locations where the strains were collected are indicated [33] . ND, not defined. Regarding 972 , locations where the strains are stocked and analyzed are indicated in parentheses. b Schematics of the SH-P sequences in strain JB22 ( 972 ) with common segments. Sequences of indicated segments exhibit 90% or higher identities with those of PomBase or 972SD4 . Black bars indicate relatively long regions that show the same segmental arrangements with those of 972SD4 and PomBase- SH2R . c Schematics of the SH-P sequences in strain JB760. Second bar shows an SH-P region of SH3L and/or SH3R of Ch3. Contigs 1–3 include SH-P regions that are not allocated to specific subtelomeres. d Schematics of the SH-P sequences in strain JB1174. C′′ is a subtype of segment C which contains six units of c motifs (see Figs. 3b and 4i ). ∆ indicates a partial sequence of each segment with no less than 10 bp decrease in total length. “?” indicates 75–90% sequence identity with the corresponding segment. e Schematics of the SH-P sequences in strain JB934. C′′′ and C′′′′, subtypes of segment C, contain seven and eight units of c motifs, respectively (see Figs. 3b and 4i ). SH1R ′ and SH2R ′ (highlighted in red) indicate that they are located at subtel2R and subtel1R in JB934, but overall sequences of telomere-side regions of Ch2R and Ch1R are homologous to those Ch1R and Ch2R in 972 , respectively (see Supplementary Fig. 4 ). Dark gray box in SH1R ′ indicates a sequence that has not been found in 972 strains and is not shared by the subtelomeres in other JB strains. f Schematics of the SH-P sequences in strain JB858. Contig 1 includes an SH-P region that is not allocated to a specific subtelomere. g Schematics of the SH-P sequences in strain JB873. Black boxes indicate common segments shared by some of JB strains, although their sequences have not been found in 972 strains (see Supplementary Fig. 5 for their sequences). Note that a partial LTR sequence is inserted at SH2L . h Schematics of the SH-P sequences in strain JB1197. i Subtypes of segment C. Note that the types of c motifs are not specified due to the relatively low reliability of sequences by long-read DNA sequencing. Full size image JB22 ( 972 ), another clone of 972 , has SH regions only at the ends of Ch1 and Ch2, not in Ch3, as in the strain 972 in our laboratory. However, SH-P regions in JB22 ( 972 ) have different segment patterns and lengths from those in 972SD4 except for SH2R , which does not contain a segment alignment homologous with PomBase- SH2R . These data indicate that chromosome rearrangement occurs frequently in SH-P regions during culturing in laboratories (Figs. 3a and 4b ). Segment patterns and lengths of SH-P regions in each 972 strain are divergent, whereas JB760, JB1174 (except for SH1R ), JB858, and JB1197 exhibit almost uniform segment patterns and lengths among the subtelomeres (Fig. 4c, d, f, h ). It is unclear which type is the original SH-P in S. pombe ; however, the divergent property is likely ancestral because repeated interchromosomal rearrangements will result in uniform patterns of SH-P regions. We detected some sequences that have not been found in 972 strains but shared by several subtelomeres in JB strains (indicated by black boxes α–δ in Fig. 4 and Supplementary Fig. 5 ). Particularly, partial sequences of SH1L and SH2R in JB873 (segments A-I-----∆P-∆Q containing black boxes) are highly homologous with the SH-P sequences in JB1197 (Fig. 4g, h ). Furthermore, JB934 does not possess any SH sequence in Ch1L , and JB873 contains partial sequence of long terminal repeat (LTR) of retrotransposon in the SH-P region of SH2L (Fig. 4e, g ). Interestingly, there are two major types of structures at chromosome ends, telomere-segment A-segment B (Tel-A-B) and telomere-partial segment F-segment G (Tel-∆F-G). Tel-A-B is found in 972 and JB760 (Figs. 3a and 4b, c ), whereas Tel-∆F-G is found in JB1174, JB934, JB858, and JB873 (Fig. 4d–g ). We found that the sequences of segments A and B is highly similar to those of partial segment F and segment G, suggesting the possibility that homologous recombination (HR) between them resulted in a Tel-∆F-G structure (Supplementary Fig. 6a ). Other possibilities are that nucleotide changes have occurred in either A-B or ∆F-G (Supplementary Fig. 6b ), or that the G-rich sequences located at the telomere-proximal ends of segment A and ∆F formed G-quadruplex-like structures and stalled replication fork progression [31] , which resulted in chromosome breakage accompanied by de novo telomere synthesis (Supplementary Figs. 3 and 6c ). Overall diversity of the SH-P regions in JB strains further support our hypothesis that SH-P regions are hot spots for genome evolution. SH-D regions in 972 strains are variable and accumulate insertions and deletions We also determined sequences of SH-D regions in 972SD4 strains by integrating the partial SH-D sequences in PomBase and our newly determined SH-D sequences. The integrated SH-D sequences were classified into common block sequences I–XI (>90% identities between the sequences of the same blocks), and supplemental homologous box sequences Ψ and Ω (Fig. 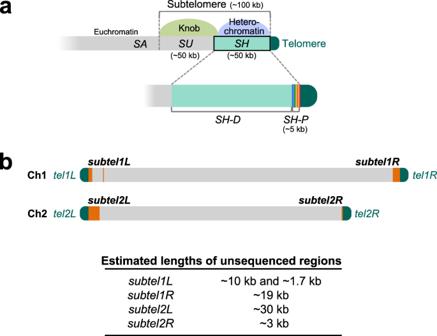Fig. 1: Structures and previously unsequenced regions of subtelomeres inS. pombe 972strain. aSchematic illustration of the structures of subtelomeres (~100 kb) of Ch1 and Ch2 in strain972. TheSHregion (~50 kb) shows high sequence identity (>90%) with other subtelomeres. Subtelomeric heterochromatin is formed around theSHregion21. AnSHsequence is composed of two characteristic regions,SH-P(~5 kb) andSH-D. In contrast, theSH-adjacentSUregion (~50 kb) shows low sequence identities with other subtelomeres, but forms a highly condensed knob structure that is shared among them24.SAindicates a subtelomere-adjacent euchromatin region.bSchematic illustration of unsequenced regions of subtelomeres in Ch1 and Ch2 of strain972according to PomBase (indicated by orange boxes).Tel1L,tel1R,tel2L, andtel2Rindicate telomeres at the left and right arms of Ch1 and those of Ch2, respectively.Subtel1L,subtel1R,subtel2L, andsubtel2Rindicate subtelomeres at the left and right arms of Ch1 and those of Ch2, respectively. Lengths of unsequenced regions are estimated based on the assumption that theseSHsequences show high similarity with that ofsubtel2Rof PomBase. Note that Ch3 is omitted in this panel (see Fig.2afor the ends of Ch3 in strain972). 5a and Supplementary Table 1 ). In contrast to the SH-P regions, the SH-D regions in strain 972 do not show duplications or differences in orders of blocks I–XI. However, we found differences in length; multiple insertions or deletions were identified in these regions (Fig. 5b ). Fig. 5: Sequence variations of SH-D regions in 972SD4 and PomBase- 972 . a Schematic illustration of homologous block (I–XI) and box (Ψ and Ω) sequences in the SH-D regions in 972SD4 and PomBase- 972 (see Supplementary Table 1 for their positions in PomBase). All SH sequences are aligned with telomeres to the left and centromeres to the right. b Comparison of SH-D regions between subtelomeres. Sequences of SH1L , SH1R , and SH2L in PomBase (indicated by green boxes) were combined with sequences newly determined in this study (yellow boxes, showing #1 clones of each SH sequence), whereas newly sequenced SH2R fragments are shown separately with PomBase- SH2R . Green and yellow numbers indicate positions in each chromosome in PomBase at the ends of overlaps between PomBase and newly determined regions. All SH sequences are aligned with telomeres to the left and centromeres to the right. Insertions (orange arrowheads) or deletions (blue arrowheads) of 10–40 bp are shown in comparison with PomBase -SH2R (thin dotted lines). Insertions and deletions of <10 bp are omitted in this panel. The thick lines connect the corresponding positions in chromosomes that are boundaries of the long regions with sequence alterations. Purple and pink boxes (Ψ) and brown, red, and orange boxes (Ω) indicate homologous sequences at the ends of the long sequence changes, 3.7 and ~7.1 kb, respectively (see Supplementary Fig. 7 for the sequences and identities between them). Numbers in black indicate chromosomal position in PomBase- SH2R . Chromosomal positions of insertions and deletions are indicated by the positions in PomBase- SH2R that are immediately before the changes (closer to the telomeres). Blue arrows in PomBase- SH2R indicate the positions of ORFs for tlh2 + and SPBCPT2R1.03 . Pale pink arrows in PomBase- SH2R indicate homologous regions (H1–5 and their inverted sequences, H1′–5′) that are utilized for chromosome fusion when telomeres are lost [53] . Gray arrows at the top indicate ranges of PCR products i–ix analyzed in c . Note that the PCR fragments i–ix in b roughly correspond to blocks I–IX in a . c Lengths of the SH-D regions in 972SD4 strains. DNA fragments i–ix were amplified by PCR using genomic DNAs of the 972 (JK107), SD5 (ST3479), and two independent 972SD4 strains (#1 and #2) as templates. Approximate DNA lengths estimated by the sequences in PomBase and 972SD4 are indicated on the right. The rap1 locus was amplified as a control. PCRs were performed at least twice. Full size image There are three big differences between subtelomeres (Fig. 5b , thick lines; note that part of them has been described in a previous study [32] ). First, there are 3.7 kb deletions in SH1R , SH2L , and SH2R at position 4,520,423 of PomBase- SH2R . Second, there is a 7.1 kb deletion in SH1R at nucleotides 4,514,836–4,507,710 of PomBase- SH2R . This deletion was detected in the three independent strains of 972SD4[1 R + ] by PFGE-Southern analysis (Fig. 2d ). Third, there is a 1.9 kb deletion in SH1L at nucleotides 4,500,309–4,498,438 of PomBase- SH2R . Intriguingly, boxes Ψ exist at the ends of the 3.7 kb change (Fig. 5a, b , purple and pink boxes, Supplementary Fig. 7a, b , and Supplementary Table 1 ). Similarly, boxes Ω exist at the ends of 7.1 kb changes (Fig. 5a, b , brown, red, and orange boxes, Supplementary Fig. 7c, d , and Supplementary Table 1 ). These data imply that the deletions and/or insertions have occurred using these homologous sequences. It is noteworthy that among Ω sequences that are indicated by different colored boxes, there are multiple insertions and deletions in the region where various repeat sequences are arranged intricately, and the sequence of ΩSH1L-L (indicated by a brown box) shows lowest sequence identity (83–85%) with other red or orange boxes (Supplementary Fig. 7c, d ). There are also smaller insertions or deletions in SH-D regions (Fig. 5b , thin dotted lines for changes of 10–40 bp compared with PomBase- SH2R ). Many of these are observed in no less than two SH-D regions, suggesting that these changes have been copied to other SH regions by chromosome rearrangement. It is also noteworthy that the newly sequenced SH2R in 972SD4[2R + ] contains an insertion at position 4,529,376 of PomBase- SH2R , indicating that this insertion has been introduced to SH2R of strain 972 in laboratories after separated from PomBase- 972 . To examine stability of the SH-D regions, their DNA structures in two independent strains of 972SD4[1 L + ] , 972SD4[1 R + ] , 972SD4[2 L + ] , and 972SD4[2 R + ] were analyzed by PCR using multiple primer sets (PCR products i–ix are indicated by gray arrows in Fig. 5b , top. Note that the fragments i–ix in Fig. 5b roughly correspond to blocks I–IX in Fig. 5a ). We found that lengths of the all PCR products matched those predicted from PomBase sequence (Fig. 5c ), indicating that the overall DNA structures of SH-D regions are stably maintained between PomBase- 972 and 972SD4 strains in contrast to those of SH-P regions. We calculated the full length of each SH region ( SH-P and SH-D ): SH1L , 61.9 kb; SH1R , 39.1 kb; SH2L , 59.1 kb; and SH2R , 49.5 kb, with SH1R having the shortest SH sequence, although these lengths are likely to change through chromosome rearrangements at SH regions. To examine evolutional change of SH-D regions, we next analyzed SH-D regions in JB strains using previous NGS data (long-read sequencing) by Tusso et al. [30] . The SH-D regions in JB22 ( 972 ) show clear differences compared with those in PomBase- 972 and 972SD4 , although the overall pattern of common blocks is very similar (Fig. 6a, b ). Block IV and a purple box (Ψ) sequences are present in both SH1L and SH2L in JB22 ( 972 ), but not in SH2L in 972SD4 . In addition, a brown box sequence (Ω) resides between blocks V and VI in SH1L and SH2L in JB22 ( 972 ), whereas the sequence is replaced by a red box sequence (Ω) in SH2L in 972SD4 . These data suggest the possibility that HR has occurred between the SH-D regions in SH1L and SH2L in JB22 ( 972 ). Thus, the SH-D regions in 972 strains are not highly stable; rather, changeable via recombination. Fig. 6: Sequence variations of SH-D regions in JB strains. a Schematic illustration of homologous block and box sequences in the SH-D regions in 972SD4 and PomBase- 972 . Note that sequences of pale blue boxes, ε–η, in the SU regions are shared by multiple subtelomeres in some of JB strains; and thus, they are defined as SH (see Fig. 6d–h , blue boxes). ORFs of the tlh genes located in block II are indicated by blue arrows. b Schematics of the SH-D sequences in strain JB22 ( 972 ) in common blocks and boxes. Sequences of indicated blocks and boxes exhibit at least 90% identities with those of PomBase- 972 . Total length of each SH-D region is indicated. c Schematics of the SH-D sequences in strain JB760. Black boxes indicate common sequences that are shared by some other JB strains but not found in 972 strains. Note that the sequence of θ is homologous with that of SAS (see main text and Supplementary Fig. 1 for the details). Contigs 1–3 are the same as those in Fig. 4c , respectively. Boxes in rainbow color [1]–[8], SH-P -like sequences; “?”, sequence with <90% identity but substantial similarity with the corresponding segment, block or box (E-value < 10 −10 in NCBI nucleotide BLAST [blastn] search); blue triangle, shorter length of the corresponding segment, block or box; gray dotted line, no sequence information available; blocks or boxes with gradation, unreliable sequence information with less than five reads. d Schematics of the SH-D sequences in strain JB1174. Inverted, opposite sequence direction from that in the corresponding block or box in 972 ; blue box, sequence shared by multiple subtelomeres as SH in some JB strains; dark gray box, sequence that has not been found in PomBase and not shared by the other JB strains; orange triangle, longer length of the corresponding block or box. e Schematics of the SH-D sequences in strain JB934. f Schematics of the SH-D sequences in strain JB858. Contig 1 is the same as that in Fig. 4f . Shaded box with red lines, an insertion of a part of mitochondrial genome. g Schematics of the SH-D sequences in strain JB873. h Schematics of the SH-D sequences in strain JB1197. Full size image SH-D regions exhibit striking variations among JB strains The SH-D regions of the other JB strains show striking variation in numbers and orders of block sequences. Furthermore, various box sequences that are not categorized as SH-D in 972 strains are shared by multiple SH-D regions in JB strains (Fig. 6c–h ). It is noteworthy that 972 strains have no SH sequence in Ch3, whereas JB760, JB1174, JB858, and JB873 possess SH-P and SH-D sequences in Ch3 (Figs. 4 and 6 ). Intriguingly, some descendent strains of 972 also possess SH sequences at either or both ends of Ch3 (Supplementary Fig. 1 , KYP33 and JP1225). These data suggest two possibilities; one is that another standard strain 975 ( h + ) contains SH sequence(s) in Ch3, and it has been transferred to descendent strains via mating and meiosis. Another is that SH regions in Ch1 or Ch2 have been translocated to Ch3 via interchromosomal recombination. In fact, the SH-P sequence in JP1225 shows high similarity with those of 972SD4 - SH2R and pNSU71 (Fig. 3a and Supplementary Fig. 1c ). However, the former is more possible because of the existence of a black box θ sequence associated with SH-D in Ch3, which has not been found in 972 strains (see below). Interestingly, multiple copies of brown box sequences (Ω) and SH-P sequences [1]–[8] are found in the SH-D sequence in JB760 (Fig. 6c ). Moreover, adjacent to block II is a black box θ. The alignment of I-II-θ is also found in Ch3 of JB1174, JB858, and JB873, although partial LTR sequences are inserted in block I in JB1174 and JB873 (Fig. 6d, f, g ). Intriguingly, the sequence of box θ is almost identical with that of SAS (spanning ~1.1 kb), which was identified as a subtelomere-associated sequence adjacent to block II in Ch3 in the descendent strains of 972 previously [21] , [27] (Supplementary Fig. 1b–d ). Thus, structures of SH-D regions in Ch3 are highly conserved in S. pombe in contrast to other parts of SH-D possibly because the ends of Ch3 are located in the nucleolus apart from those of Ch1 and Ch2 located in the nucleus in vegetatively growing cells [17] , which may restrain interchromosomal recombination between Ch3 and Ch1 or Ch2. The SH-D regions of JB strains except for JB22 ( 972 ) and JB760 showed high variation in their compositions and lengths; however, they share some common features. (1) Blocks I and II are highly conserved. (2) Multiple copies of parts of the SU regions in 972 (indicated by pale blue boxes, ε–η, in Fig. 6a , see Supplementary Table 1 for their positions) are found in the SH regions in these strains (indicated by blue boxes in Fig. 6 ). (3) Multiple black boxes, θ–τ, which are not found in 972 are also shared by the subtelomeres of JB strains except for JB22 ( 972 ) (Fig. 6 ). (4) Blocks I and XI (green) and boxes ε (blue) and ζ (blue) are found inverted compared with those in 972 (Fig. 6d, e, g ). (5) Surprisingly, the SU region of JB858 and the SH-D regions of JB858 and JB873 contain sequences of parts of mitochondrial genome (indicated by Mt in Fig. 6f, g ). The overall changes in SH-D regions in JB strains indicate that complexed chromosome rearrangements have occurred in the course of evolution of S. pombe even after strain 972 has been isolated. Subtelomeres are hot spots for mutations Given that the SH-P regions of 972SD4 contain multiple nucleotide changes compared with those in PomBase- 972 (Fig. 3 and Supplementary Fig. 3 ), we examined whether mutation rates are specifically high in subtelomeres. First, sequences of multiple loci in the SH-D of SH2R in two independent 972SD4[2 R + ] strains (#1 and #2) were determined and compared with those of PomBase- 972 (Fig. 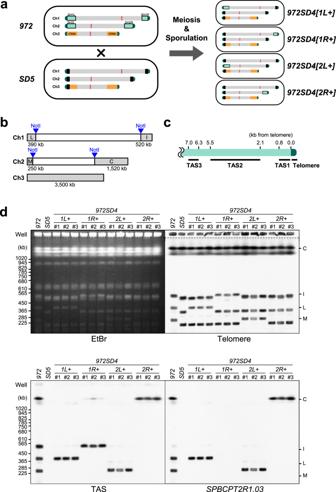Fig. 2: Construction of972SD4strains containing a singleSHregion of strain972. aConstruction strategy of972SD4strains. Pale green boxes,SHregions adjacent to telomeres; black boxes, marker genes (his7+orura4+) that replacedSHregions21; orange boxes, rDNA repeats; and red boxes, centromeres. Strains972andSD5were crossed, and meiosis and sporulation (spore formation) were induced. Progeny with singleSHregions were obtained.bSchematic illustration of telomere-containing NotI restriction fragments (shown in gray). Fragments L, I, M, and C containSH1L,SH1R,SH2L, andSH2R, respectively. The size of each fragment is shown underneath.cSchematic illustration of the positions of DNA fragments detected by probes for telomeres and TAS (TAS1–3). Shown are the distances from telomeres in pNSU70.dAnalyses of the chromosome end structures in972SD4strains. NotI-digested chromosomal DNAs of three independent strains of each972SD4were analyzed by PFGE followed by Southern blotting using telomere, TAS, orSPBCPT2R1.03ORF probes. EtBr, ethidium bromide staining of the gel after PFGE. Note thatSH1Rlacks part of theSHregion homologous toSPBCPT2R1.03according to PomBase. Consistently,972SD4[1R+]strains did not show anSPBCPT2R1.03. signal (also see Fig.5). These data were reproduced twice. 7 and Supplementary Table 2 ). We found that regions around the tlh2 gene locus exhibit high rates of mutations. Most of them are point mutations, but some are changes of numbers of repeat sequences, such as [T] n . It should be noted that the two 972SD4[2 R + ] strains possess different sequences in the tlh2 locus (99.44% vs. 99.41% identities with PomBase). In contrast, the telomere-distal half of SH-D region and all chromosomal regions outside of SH , i.e., the SU region, the subtelomere boundary region, the SA region (see Fig. 1a ), and various gene loci in Ch1 or Ch2 in the two 972SD4[2R + ] strains show 100% sequence identities with those in PomBase- 972 , indicating strict preservation of their DNA sequences through repeated rounds of cell division. These data suggest that the telomere-proximal half of SH-D regions (~20 kb), as well as SH-P regions are particularly prone to the accumulation of mutations. Fig. 7: Subtelomeres are hot spots for sequence variation. Sequence identities between PomBase- 972 and other S. pombe strains used in this study. Sequences of the SH-D and SU regions, the subtelomere boundary, and the SA region in Ch2R , and those of other gene loci of three categories were analyzed (see Supplementary Table 2 for the details). Note that two independent 972SD4[2 R + ] strains (clones #1 and #2) contain different sequences around the tlh2 gene locus. Full size image We next examined mutation rates in JB strains using previous NGS data (long-read sequencing by Tusso et al. [30] and short-read sequencing with high accuracy using Illumina HiSeq 2000 by Jeffares et al. [33] , see “Methods” section for details). Only the chromosomal loci outside of SH were analyzed because SH regions are not distinguishable using short reads. We found that JB22 ( 972 ) showed 100% sequence identities with PomBase- 972 at the all loci examined (Fig. 7 and Supplementary Table 2 ), indicating that genome integrity is strictly maintained through repeated rounds of cell division at these loci. In striking contrast, JB strains other than JB22 ( 972 ) exhibit high mutation rates at the SU , subtelomere boundary, and SA regions in Ch2R (Fig. 7 and Supplementary Table 2 ), indicating that subtelomeres are prone to nucleotide changes during the long-time course of S. pombe evolution. Interestingly, some JB strains show relatively high mutation rates at the chromosome loci of nonessential genes, especially the rap1 gene (Fig. 7 and Supplementary Table 2 ). Rap1 is a subunit of the shelterin complex, which protects chromosome ends and regulates various telomere functions [15] , [34] . Rap1 is recruited to telomeres partly through interaction with a telomere DNA-binding protein Taz1 and associates with multiple proteins to regulate various telomere functions [34] , [35] , [36] . Amino acid changes of Rap1 are rarely found in the regions for interactions with its partners (Supplementary Fig. 8 ). We found one amino acid change, glutamic acid (E) 671 to arginine, in the RCT (Rap1 C-terminal) domain of Rap1, which mediates interaction of Rap1 with Taz1; however, it was suggested that E671 is not involved in their direct interaction [37] . Moreover, one amino acid change, E424 to alanine, is found in the DD (dimerization domain) of Taz1, which is important for Taz1 binding to telomere DNA; however, E424 is located outside of the direct interaction domain [38] . Furthermore, we found that the sequences of telomere repeats in JB strains are highly similar to those in 972 strains. Thus, it seems that the principal functions of Rap1 and Taz1 are conserved during the course of S. pombe evolution. It is likely that the higher mutation rates in the rap1 and taz1 genes are because their gene products are more tolerant to amino acid changes than other gene products. Identification of additional members of the subtelomeric RecQ helicase gene family In genome sequences in PomBase -972 , there are two RecQ helicase genes, tlh1 (partial) and tlh2 , which have been allocated to SH1L and SH2R , respectively. Parts of the DNA sequences of tlh1/2 are homologous with the dh repeat sequence of pericentromeres and serve as templates for small interfering RNA (siRNA) produced by RNA interference (RNAi) machinery; further, the siRNA participates in the initiation of subtelomeric heterochromatin formation [22] , [23] . Our sequencing data of SH regions newly identified two members of the tlh gene family, tlh3 and tlh4 , in SH1R and SH2L , respectively. Thus, genome of strain 972 contains four tlh genes in total (Fig. 8a and Supplementary Fig. 9 ). Fig. 8: Identification of tlh genes with multiple mutations. a Identification of tlh3 and tlh4 . Chromosomal locations of the four tlh genes are shown. b Summary of predicted ORFs and nucleotide changes in the tlh genes of 972SD4 compared with the tlh2 gene in PomBase. The top panel shows the tlh2 locus in PomBase. Seven digit numbers indicate chromosomal positions on Ch2 in PomBase. Blue arrow with a purple line, the tlh2 ORF defined in PomBase; brown bar, dh -homologous region; light purple line, predicted coding region which is in-frame with that of the tlh2 ORF in PomBase; light or dark green line, predicted coding region in the reading frame different from that of the predicted tlh2 ORF in PomBase; yellow star, point mutation (no frame shift); orange arrowhead, nucleotide insertion (numbers of inserted nucleotides are shown below); blue arrowhead, nucleotide deletion (numbers of deleted nucleotides are shown below); dM the original first methionine codon of the tlh2 ORF in PomBase, uM putative first methionine codon upstream of dM for PomBase- tlh2 , uM′ putative first methionine codon for the short ORF, dM′ putative first methionine codon for the long ORF, T termination codon. c Expression of RNA of the dh -homologous region in the tlh genes in strains 972 , SD5 , and 972SD4 in a clr4 ∆ background was analyzed by quantitative RT-PCR in the presence (+) or absence (−) of RNase. Expression level of tlh + relative to that of his1 + was normalized to that in 972 (−RNase). Data are presented as mean values ± SD (standard deviations). N = 3 biologically independent experiments (each value is indicated by a gray dot). Full size image The descendent strains of 972 possess additional tlh ORF(s) in Ch3 (Supplementary Fig. 1 ), that may have transferred from their other chromosome ends or from mating partners. We also found multiple putative tlh genes in the SH-D regions of JB strains (Fig. 6 , blue arrows). All JB strains possess at least two tlh genes because tlh genes are located in block II, which is highly conserved among the strains. The tlh genes contain multiple nucleotide changes Examination of the tlh sequences raised the possibility that the ORF for the tlh2 gene is not properly defined in PomBase. In the sequence of PomBase- SH2R , there is an in-frame methionine (Met) codon (uMet [ u pstream Met ]) 543 bases (corresponding to 181 amino acids) upstream of the original first Met codon (dMet [ d ownstream Met ]) that was defined by PomBase (Fig. 8b and Supplementary Fig. 9 ). The sequences surrounding these Met codons match the Kozak consensus sequence (A/GNN ATG G, the initiation codon underlined), which participates in the initiation of translation in eukaryotes [39] , suggesting that the uMet may be the true initiation codon for translation. Unexpectedly, each of the newly sequenced tlh1–4 genes of 972SD4 was found to contain multiple nucleotide changes (i.e., point mutations, insertions, and deletions) compared with the tlh2 gene in PomBase (Fig. 8b and Supplementary Fig. 9 ). There are tandem repeat sequences at the loci where insertion occurred in the long coding region: [ATGACA] n at the most N-terminal insertion (the 6 bp insertion), [CGACAA] n at the middle insertion (the 18 or 24 bp insertion), and [TGATGG] n at the most C-terminal insertion (the 6 bp insertion), suggesting that these repetitive sequences are highly prone to recombination (Fig. 8b , orange arrowheads). Because of these changes, the uMet′ codons of tlh1 , tlh2 , and tlh4 located upstream of uMet are no longer in-frame to the long coding sequence from the dMet codons, and only short coding sequences are predicted because of a termination codon derived by a point mutation (Fig. 8b , light purple lines with a dark green line). Intriguingly, multiple nucleotide changes, including point mutations, insertions, and deletions, did not introduce premature termination codons within the long ORFs of the tlh genes in 972SD4 . Similarly, the tlh gene(s) of Ch3 in the 972 descendent strains (KYP33 and JP1225) lack 24 bp immediate downstream of the dMet codons; however, no frame shift occurs, and uMet′ codons are supplied by the SAS sequence in the same codon frame (Supplementary Fig. 1d ). RNA expression from the tlh genes in 972SD4 To examine our assumption that the tlh genes have longer protein-coding sequence than that previously predicted by PomBase, we determined ranges of tlh RNA expression by reverse transcription (RT)-PCR (Supplementary Fig. 10 ). We detected RNAs of tlh genes that contain at least 950 bases upstream of the dMet codon (~400 bp upstream of the uMet codon). These data suggest that the tlh genes may have protein-coding sequences that are potentially 543 bases longer than that defined in PomBase (Fig. 8b , a light purple line in the top panel). To examine whether the tlh genes in 972SD4 carrying multiple mutations are capable to produce dh RNAs that participate in the formation of subtelomeric heterochromatin, we determined the RNA expression level from the dh -homologous region of each tlh gene in clr4 ∆ cells where the strong gene silencing by subtelomeric heterochromatin is omitted [23] . We found that these four tlh genes express dh RNAs; however, the expression levels were lower than one-fourth of that in the wild-type strain possibly due to lack of positive feedback regulation by other tlh RNA expression (Fig. 8c ). These results suggest that DNAs of the tlh genes are prone to mutations without severely affecting RNA expression. This study describes in-depth analyses of subtelomeres in S. pombe . We obtained complete sequences of subtelomeres in the standard S. pombe strain 972 by producing strains with single SH regions. We also extracted SH sequences of some natural isolates of S. pombe strains (JB strains) from previous NGS data. The whole sequences revealed that SH regions are composed of two parts: the telomere-adjacent SH-P region and telomere-distal SH-D region. The SH-P region is a mosaic of multiple common segments that vary among subtelomeres and strains, suggesting that this region is highly prone to chromosomal rearrangement during cell divisions. In contrast, the SH-D region shows high sequence similarity among subtelomeres and 972 strains, although there are some insertions, deletions, and chromosomal rearrangement, suggesting that the overall DNA structure of this region is stably maintained during short-term culturing. However, JB strains other than JB22 ( 972 ) exhibited striking variation in the structures of SH-D regions, indicating that SH-D regions are also susceptible to chromosomal rearrangement during long-term evolution of S. pombe . Interestingly, not only SH but also SU regions exhibit high rates of nucleotide changes among strains, whereas chromosomal regions outside of this region are subject to highly strict genome preservation. Thus, subtelomeres are hot spots for genome evolution and exhibit multiple patterns of genome variation (Fig. 9 ). Fig. 9: Summary of features of S. pombe subtelomeres. The S. pombe SH region is composed of two parts: the SH-P region with a mosaic of multiple segments, and the SH-D region with multiple blocks and boxes containing deletions and insertions. Colors of bars indicate relative rates of chromosome rearrangement or nucleotide alteration versus PomBase (orange, high rate; blue, low rate). The SH-P region shows high rates of chromosome rearrangement and nucleotide alteration even between the 972 strains ( 972SD4 and JB22 vs. PomBase), whereas the SH-D region shows lower rates of these changes compared with those in the SH-P region. The SU , boundary, and SA regions and the rap1 and taz1 loci also exhibit medium levels of these changes in the JB strains that are phylogenetically distant from 972 . Thus, chromosomal regions around the subtelomeres (and the rap1 and taz1 loci) are prone to genome diversity. Dotted line indicates a region that was unable to be analyzed with the NGS data. Full size image Human subtelomeres ( SH regions in humans) are also mosaics of multiple common segments that correspond to the SH-P region in S. pombe . However, they contain no sequence equivalent to that of the SH-D region, i.e., a relatively long common sequence shared by all subtelomeres [9] , [19] . Common segments of the same categories are mostly nonidentical (~90–100% identities), and the location and copy number of each segment vary among individuals [9] , [40] . In S. cerevisiae , the subtelomeres have common X and Y′ elements, and ORFs of proteins such as PAU and FLO families; however, copy numbers of the Y′ element and the ORFs are highly variable among strains [18] , [41] . Based on these findings and studies in other species, along with our results in S. pombe , we propose that high variation in SH sequences is a common feature in eukaryotes. What underlies this high variation of SH regions? First, DNA double-strand breaks (DSBs) are repaired by either HR or nonhomologous end joining. Vegetative cell cycle of the wild-type S. pombe strain lacks G 1 phase because cells already possess sufficient mass to proceed to S phase when the previous mitosis is completed. Therefore, ~80% period of the S. pombe cell cycle is G 2 phase, when HR predominates for DSB repair [42] . Because of the high sequence identities among SH regions, DNA repair by HR may occur frequently between SH regions of different chromosomes (interchromosomal repairs), as well as between sister chromosomes (intrachromosomal repairs), which causes gross rearrangement of chromosomes. Second, repetitive sequences within SH regions may be recognized by HR machineries, causing amplification or deletion of the repeat units. Third, repetitive sequences, including S. pombe telomeres and subtelomeres, are regions intrinsically difficult to replicate during S phase [43] , [44] , [45] . Replication fork collapse and erosion of telomeres and subtelomeres can result in formation of single-ended DNA breaks that are repaired by break-induced replication (BIR) [46] . Recent studies suggested that BIR is a highly inaccurate DNA repair mechanism, and causes high levels of mutations and chromosome rearrangements [47] , [48] , [49] , [50] , [51] , [52] . Therefore, BIR may cause high rates of mutations and chromosome rearrangements in SH regions. Fourth, the SH-D region serve as a fusion point of chromosome circularization when telomeres are lost [53] . S. pombe has only three chromosomes, which enables cells to survive telomere crisis by self-circularization of each chromosome [29] . Chromosome end fusions of Ch1 and Ch2 take place between H1–5 and their inverted sequences, H1′–5′, which are located in blocks I, II, and V (Fig. 5b , pink arrows) [53] . It is possible that chromosome circularization and re-linearization promote chromosome rearrangement of SH-D regions. Importantly, in the subtelomeres (i.e., the SH and SU regions) of S. pombe , there is no gene essential for cell growth under normal culture conditions, and deletion of all SH regions does not affect cell growth per se [21] . Genomes of other species also contain multiple copies of the same genes in SH regions. This may explain why cells can continue to grow, even with mutations in SH (and SU ) regions, resulting in the accumulation of mutations. The SU regions are known to form knob bodies that are highly condensed chromatin structures, which may prevent precise DNA replication or normal DNA repair, and causes the accumulation of nucleotide alterations [21] , [24] (Fig. 9 ). Surprisingly, the tlh genes in 972SD4 contain no nonsense mutation in their ORFs, although they contained various mutations compared with the tlh2 gene in PomBase. We found that some of the mutations cause alterations in the amino acid sequences of the conserved RecQ motif (Supplementary Fig. 11 ). Absence of premature termination codon is important for suppression of mRNA degradation mediated by the NMD (nonsense-mediated mRNA decay) mechanism [54] . Thus, it is likely that the principal function of the tlh genes is to produce RNAs containing dh sequences, and that presence of the tlh ORFs is advantageous for their normal RNA expression, which induces heterochromatin formation. Although a previous study suggested that the tlh genes are involved in survival after telomere shortening [55] , functions of the Tlh protein is not clarified yet. Over 70 years since Dr. Urs Leupold isolated S. pombe standard strains, 968 ( h 90 ), 972 ( h − ), and 975 ( h + ), from the Delft culture [26] , it has been believed that these three strains possess almost the same genetic information except for the mating-type genes. This and previous studies have shown that 972 has no SH sequence in Ch3, whereas some of its descendent strains possess SH region(s) with SAS in Ch3 [21] , [27] , [28] (Fig. 6 and Supplementary Fig. 1 ). It is noteworthy that the SAS sequence is absent from the genome of 972 . The three standard strains have been traveling over the world to produce numerous number of descendent strains through mating and meiosis [56] . Therefore, the assumption is that 968 and/or 975 had already had SH region(s) in Ch3 when they were first isolated. Taken together, we propose that subtelomeres are highly polymorphic chromosomal regions and contribute to genome evolution. In this study, we have shown that the DNA sequence of the tlh2 gene has changed from that of the original strain 972 after repeated rounds of cell division (Fig. 8b ). Human SH regions also contain various genes, such as DUX4 (associated with facioscapulohumeral muscular dystrophy) and olfactory receptor genes [9] , [19] . Thus, the high rates of polymorphisms in SH regions may contribute to human diversity and sometimes to disease susceptibilities. It is intriguing to investigate correlation between various human diseases and SH sequences. Overall, genome rearrangement, deletion, insertion, and mutation can cause changes in ORFs, which may result in diversification of species. 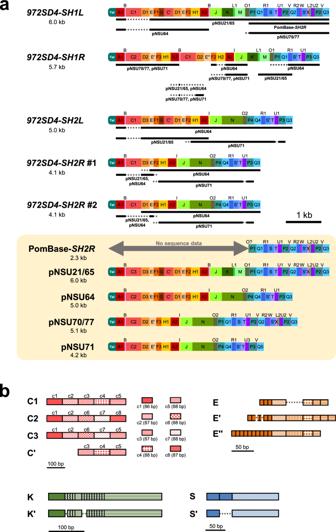Fig. 3: Highly variableSH-Pregions consist of common segments in strain972. aSchematics ofSH-Pregions. TheSH-Psequences were classified into common segments (A–X) and their variants (see Supplementary Fig.3for each sequence).SH-Pregions of972SD4strains, a partialSH2Rregion in PomBase (PomBase-SH2R), andSH-Pregions of a pNSU series in PomBase are shown. The total length of eachSH-Pregion is indicated. Note that972SD4-SH1L,972SD4-SH1R, and972SD4-SH2Lobtained from two independent972SD4strains (i.e., #1 and #2 clones) are identical, whereas972SD4-SH2R#1 and #2 contain different variants D, D1 and D3. Black bars indicate relatively long regions that show the same segments and variants with those of pNSUs or PomBase-SH2R, whereas gray dotted lines indicate regions that show the same segments but different variants.bSubtypes of C, E, K, and S consist of common sequence motifs with different copy numbers. The boxes with the same color and pattern show 100% sequence identity. Segment C consists of three variants, C1–3, that are composed of homologous sequence motifs, c1–8, that show >82% identities with each other (see Supplementary Fig.3c, c*for details). Strains and general techniques for S. pombe S. pombe strains used in this study are listed in Supplementary Table 3 . Growth media and basic genetic and biochemical techniques used in this study were described previously [57] , [58] , [59] . Construction of 972SD4 strains To construct 972SD4 strains carrying single SH regions of the standard wild-type strain 972 , the SD5 strain (ST3524) [21] , in which all five SH regions were replaced with selective marker genes ( his7 + or ura4 + ), was crossed with strain 972 , and then the progeny were crossed back with the SD5 strain (ST3479 or ST3524) again. The presence or absence of each SH region in the resulting progeny were examined by PFGE followed by Southern blotting. PFGE PFGE of NotI-digested chromosomal DNA was performed using a CHEF-DR III Pulsed-Field Electrophoresis System (BioRad) under the following conditions: 1% SeaKem Gold Agarose (Lonza) in 0.5× TBE; temperature, 10 °C; initial switch time, 40 s; final switch time, 80 s; run time, 18 h; voltage gradient, 6.8 V/cm; and angle, 120°. Southern blotting NotI-digested chromosomal DNA was separated by PFGE and subjected to Southern blotting. Telomeric DNA and TAS fragments (TAS1, TAS2, and TAS3) were excised from pNSU70 [25] , and used as the telomere and TAS probes, respectively. The SPBCPT2R1.03 ORF was amplified by PCR and used as the probe that specifically recognizes the SH-D regions of subtel1L , subtel2L , and subtel2R , but not subtel1R in 972 . These DNA fragments were labeled with digoxigenin (DIG), using a DIG High Prime DNA Labeling and Detection Starter Kit II (Roche), and signals were detected according to the manufacturer’s instructions. Cloning and sequencing of SH regions DNA fragments containing SH-P regions (~5 kb) were amplified by PCR from genomic DNA of each 972SD4 strain using Phusion High-Fidelity DNA polymerase (Thermo Fisher) and the following primers. jk1861:5^'- ACTAGTGGATCCCCCTGTAACCACGTAACCTTGTAACC - 3^'
 
    jk1862:5^' - GAATTCCTGCAGCCCGGTTTGAGCATCTGTCAGAGGTAA - 3^'
 Each DNA fragment was inserted at the Sma1 site of pBluescript SK(−) (Stratagene) using In-Fusion HD Cloning Kit (Clontech). The resulting plasmids were digested with Kpn1 and Xho1 at the multiple cloning site of the vector and treated with exonuclease III (Takara) and mung bean nuclease (Takara) for fixed times to obtain deletion series from the XhoI cutting site (5′-protruding end). Both ends of the plasmids were blunted with Klenow fragments (Takara) and ligated with DNA ligase (Takara). The re-circularized plasmids were cloned using E. coli , XL1-Blue ( recA1 endA1 gyrA96 thi-1 hsdR17 supE44 relA1 lac [F′ proAB lacI q Z ∆ M15 Tn 10 (Tet r )]), and then sequenced using the following primers that anneal to the vector. st13 ( M13 primer M3):5^'- GTAAAACGACGGCCAGT - 3^'
 
    st14 ( M13 primer RV):5^' - CAGGAAACAGCTATGAC - 3^'
 The DNA sequence of SH-P was assembled using the overlapping sequences of serial deletion plasmids (Supplementary Fig. 2 ). Two independent strains of each 972SD4 were analyzed. DNA fragments (1.3–2.9 kb) of the SH-D region were amplified by PCR and sequenced, except for the regions with some repeats that were sequenced using the deletion method described above. Two independent strains of each 972SD4 were analyzed. DNA sequences were determined using BigDye Terminator v3.1 Cycle Sequencing Kit (Applied Biosystems), Prism 3130 xl Genetic Analyzer (Applied Biosystems), and DNA Sequencing Analysis Software v5.4 (Applied Biosystems). In addition, some DNA sequences were determined by Eurofins Genomics Inc. Analyses of previous NGS data of JB strains To analyze DNA sequences at subtelomeres and other chromosomal loci in JB strains, we utilized previous raw data from NGS by Tusso et al. (long-read sequencing by Nanopore MinION and PacBio RS II; NCBI Sequence Read Archive, PRJNA527756 [ https://www.ncbi.nlm.nih.gov/bioproject/PRJNA527756 ]) [30] and those by Jeffares et al. (short-read sequencing by Illumina HiSeq 2000; European Nucleotide Archive, PRJEB2733 [ https://www.ebi.ac.uk/ena/browser/view/PRJEB2733 ]) [33] . De novo assembly of the long reads (by MinION) were performed as follows. Adaptor and its adjacent (10–20 bp) sequences in raw read data were trimmed using Porechop (v0.2.4, https://github.com/rrwick/Porechop ) and fastp (v0.20.1) [60] . The trimmed long reads were assembled by Canu 2.0 (ref. [61] ), using the NIG supercomputer. Chromosome configurations compared with those in strain 972 were analyzed using MUMmer4 (ref. [62] ). To determine sequences at SH regions, we collected long reads that contain telomere repeats and telomere-adjacent segments at their ends using NCBI nucleotide BLAST (blastn). The collected reads were classified into several categories using AliView (v1.26) [63] and MAFFT (v7.453) [64] , and the sequences of each category were combined into one consensus sequence using Minimap2 (v.2.17-r941) [65] and Racon (v1.4.13) [66] . Locations of the SH sequences were determined by search for homologous sequences in the chromosome assembly described above. Long-read data (by PacBio RS II) were also used to improve the quality of sequences. To determine sequences other than SH , we searched target sequences in the de novo assembly described above and polished them by Pilon (v1.23) [67] using short-read data. RNA analyses Total RNA was purified from exponentially growing cells as described previously [28] . For the RT-PCR, complementary DNA was synthesized with random primers using a High-Capacity cDNA Reverse Transcription Kit (Applied Biosystems) and analyzed by conventional PCR (Supplementary Fig. 10 ) or quantitative PCR using a StepOne Real-Time PCR System (Fig. 8c ). 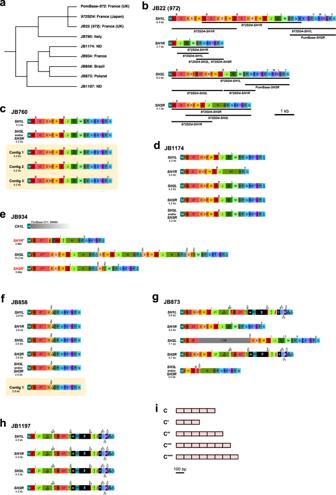Fig. 4: High variation inSH-Pregions in diverseS. pombestrains. aPhylogenetic relationships among972and JB strains based on genome-wide sequences according to a previous study by Tusso et al.30. Locations where the strains were collected are indicated33. ND, not defined. Regarding972, locations where the strains are stocked and analyzed are indicated in parentheses.bSchematics of theSH-Psequences in strain JB22 (972) with common segments. Sequences of indicated segments exhibit 90% or higher identities with those of PomBase or972SD4. Black bars indicate relatively long regions that show the same segmental arrangements with those of972SD4and PomBase-SH2R.cSchematics of theSH-Psequences in strain JB760. Second bar shows anSH-Pregion ofSH3Land/orSH3Rof Ch3. Contigs 1–3 includeSH-Pregions that are not allocated to specific subtelomeres.dSchematics of theSH-Psequences in strain JB1174. C′′ is a subtype of segment C which contains six units of c motifs (see Figs.3band4i). ∆ indicates a partial sequence of each segment with no less than 10 bp decrease in total length. “?” indicates 75–90% sequence identity with the corresponding segment.eSchematics of theSH-Psequences in strain JB934. C′′′ and C′′′′, subtypes of segment C, contain seven and eight units of c motifs, respectively (see Figs.3band4i).SH1R′ andSH2R′ (highlighted in red) indicate that they are located atsubtel2Randsubtel1Rin JB934, but overall sequences of telomere-side regions ofCh2RandCh1Rare homologous to thoseCh1RandCh2Rin972, respectively (see Supplementary Fig.4). Dark gray box inSH1R′ indicates a sequence that has not been found in972strains and is not shared by the subtelomeres in other JB strains.fSchematics of theSH-Psequences in strain JB858. Contig 1 includes anSH-Pregion that is not allocated to a specific subtelomere.gSchematics of theSH-Psequences in strain JB873. Black boxes indicate common segments shared by some of JB strains, although their sequences have not been found in972strains (see Supplementary Fig.5for their sequences). Note that a partial LTR sequence is inserted atSH2L.hSchematics of theSH-Psequences in strain JB1197.iSubtypes of segment C. Note that the types of c motifs are not specified due to the relatively low reliability of sequences by long-read DNA sequencing. 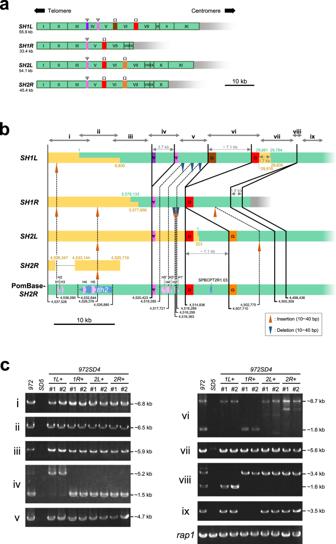Fig. 5: Sequence variations ofSH-Dregions in972SD4and PomBase-972. aSchematic illustration of homologous block (I–XI) and box (Ψ and Ω) sequences in theSH-Dregions in972SD4and PomBase-972(see Supplementary Table1for their positions in PomBase). AllSHsequences are aligned with telomeres to the left and centromeres to the right.bComparison ofSH-Dregions between subtelomeres. Sequences ofSH1L,SH1R, andSH2Lin PomBase (indicated by green boxes) were combined with sequences newly determined in this study (yellow boxes, showing #1 clones of eachSHsequence), whereas newly sequencedSH2Rfragments are shown separately with PomBase-SH2R. Green and yellow numbers indicate positions in each chromosome in PomBase at the ends of overlaps between PomBase and newly determined regions. AllSHsequences are aligned with telomeres to the left and centromeres to the right. Insertions (orange arrowheads) or deletions (blue arrowheads) of 10–40 bp are shown in comparison with PomBase-SH2R(thin dotted lines). Insertions and deletions of <10 bp are omitted in this panel. The thick lines connect the corresponding positions in chromosomes that are boundaries of the long regions with sequence alterations. Purple and pink boxes (Ψ) and brown, red, and orange boxes (Ω) indicate homologous sequences at the ends of the long sequence changes, 3.7 and ~7.1 kb, respectively (see Supplementary Fig.7for the sequences and identities between them). Numbers in black indicate chromosomal position in PomBase-SH2R. Chromosomal positions of insertions and deletions are indicated by the positions in PomBase-SH2Rthat are immediately before the changes (closer to the telomeres). Blue arrows in PomBase-SH2Rindicate the positions of ORFs fortlh2+andSPBCPT2R1.03. Pale pink arrows in PomBase-SH2Rindicate homologous regions (H1–5 and their inverted sequences, H1′–5′) that are utilized for chromosome fusion when telomeres are lost53. Gray arrows at the top indicate ranges of PCR products i–ix analyzed inc. Note that the PCR fragments i–ix inbroughly correspond to blocks I–IX ina.cLengths of theSH-Dregions in972SD4strains. DNA fragments i–ix were amplified by PCR using genomic DNAs of the972(JK107),SD5(ST3479), and two independent972SD4strains (#1 and #2) as templates. Approximate DNA lengths estimated by the sequences in PomBase and972SD4are indicated on the right. Therap1locus was amplified as a control. PCRs were performed at least twice. Primer sequences are listed in Supplementary Table 4 . 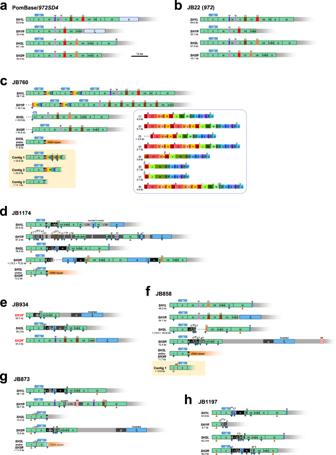Fig. 6: Sequence variations ofSH-Dregions in JB strains. aSchematic illustration of homologous block and box sequences in theSH-Dregions in972SD4and PomBase-972. Note that sequences of pale blue boxes, ε–η, in theSUregions are shared by multiple subtelomeres in some of JB strains; and thus, they are defined asSH(see Fig.6d–h, blue boxes). ORFs of thetlhgenes located in block II are indicated by blue arrows.bSchematics of theSH-Dsequences in strain JB22 (972) in common blocks and boxes. Sequences of indicated blocks and boxes exhibit at least 90% identities with those of PomBase-972. Total length of eachSH-Dregion is indicated.cSchematics of theSH-Dsequences in strain JB760. Black boxes indicate common sequences that are shared by some other JB strains but not found in972strains. Note that the sequence of θ is homologous with that of SAS (see main text and Supplementary Fig.1for the details). Contigs 1–3 are the same as those in Fig.4c, respectively. Boxes in rainbow color [1]–[8],SH-P-like sequences; “?”, sequence with <90% identity but substantial similarity with the corresponding segment, block or box (E-value < 10−10in NCBI nucleotide BLAST [blastn] search); blue triangle, shorter length of the corresponding segment, block or box; gray dotted line, no sequence information available; blocks or boxes with gradation, unreliable sequence information with less than five reads.dSchematics of theSH-Dsequences in strain JB1174. Inverted, opposite sequence direction from that in the corresponding block or box in972; blue box, sequence shared by multiple subtelomeres asSHin some JB strains; dark gray box, sequence that has not been found in PomBase and not shared by the other JB strains; orange triangle, longer length of the corresponding block or box.eSchematics of theSH-Dsequences in strain JB934.fSchematics of theSH-Dsequences in strain JB858. Contig 1 is the same as that in Fig.4f. Shaded box with red lines, an insertion of a part of mitochondrial genome.gSchematics of theSH-Dsequences in strain JB873.hSchematics of theSH-Dsequences in strain JB1197. 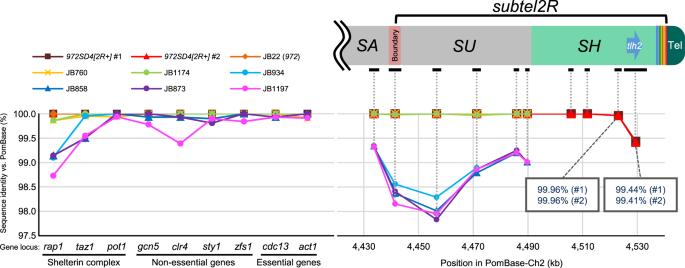Fig. 7: Subtelomeres are hot spots for sequence variation. Sequence identities between PomBase-972and otherS. pombestrains used in this study. Sequences of theSH-DandSUregions, the subtelomere boundary, and theSAregion inCh2R, and those of other gene loci of three categories were analyzed (see Supplementary Table2for the details). Note that two independent972SD4[2R+]strains (clones #1 and #2) contain different sequences around thetlh2gene locus. 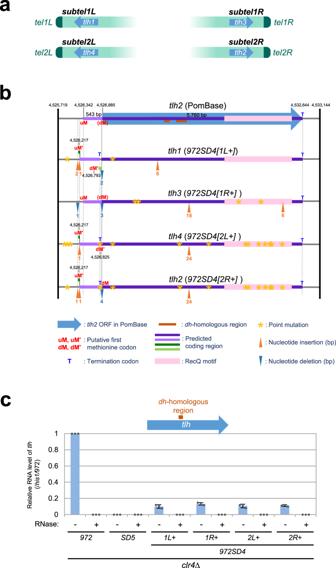Fig. 8: Identification oftlhgenes with multiple mutations. aIdentification oftlh3andtlh4. Chromosomal locations of the fourtlhgenes are shown.bSummary of predicted ORFs and nucleotide changes in thetlhgenes of972SD4compared with thetlh2gene in PomBase. The top panel shows thetlh2locus in PomBase. Seven digit numbers indicate chromosomal positions on Ch2 in PomBase. Blue arrow with a purple line, thetlh2ORF defined in PomBase; brown bar,dh-homologous region; light purple line, predicted coding region which is in-frame with that of thetlh2ORF in PomBase; light or dark green line, predicted coding region in the reading frame different from that of the predictedtlh2ORF in PomBase; yellow star, point mutation (no frame shift); orange arrowhead, nucleotide insertion (numbers of inserted nucleotides are shown below); blue arrowhead, nucleotide deletion (numbers of deleted nucleotides are shown below); dM the original first methionine codon of thetlh2ORF in PomBase, uM putative first methionine codon upstream of dM for PomBase-tlh2, uM′ putative first methionine codon for the short ORF, dM′ putative first methionine codon for the long ORF, T termination codon.cExpression of RNA of thedh-homologous region in thetlhgenes in strains972,SD5, and972SD4in aclr4∆ background was analyzed by quantitative RT-PCR in the presence (+) or absence (−) of RNase. Expression level oftlh+relative to that ofhis1+was normalized to that in972(−RNase). Data are presented as mean values ± SD (standard deviations).N= 3 biologically independent experiments (each value is indicated by a gray dot). 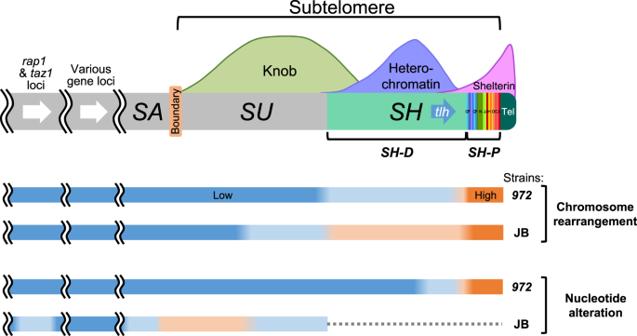Fig. 9: Summary of features ofS. pombesubtelomeres. TheS. pombe SHregion is composed of two parts: theSH-Pregion with a mosaic of multiple segments, and theSH-Dregion with multiple blocks and boxes containing deletions and insertions. Colors of bars indicate relative rates of chromosome rearrangement or nucleotide alteration versus PomBase (orange, high rate; blue, low rate). TheSH-Pregion shows high rates of chromosome rearrangement and nucleotide alteration even between the972strains (972SD4and JB22 vs. PomBase), whereas theSH-Dregion shows lower rates of these changes compared with those in theSH-Pregion. TheSU, boundary, andSAregions and therap1andtaz1loci also exhibit medium levels of these changes in the JB strains that are phylogenetically distant from972. Thus, chromosomal regions around the subtelomeres (and therap1andtaz1loci) are prone to genome diversity. Dotted line indicates a region that was unable to be analyzed with the NGS data. Reporting summary Further information on research design is available in the Nature Research Reporting Summary linked to this article.